Rydberg atoms in hollow-core photonic crystal fibres The exceptionally large polarizability of highly excited Rydberg atoms—six orders of magnitude higher than ground-state atoms—makes them of great interest in fields such as quantum optics, quantum computing, quantum simulation and metrology. However, if they are to be used routinely in applications, a major requirement is their integration into technically feasible, miniaturized devices. Here we show that a Rydberg medium based on room temperature caesium vapour can be confined in broadband-guiding kagome-style hollow-core photonic crystal fibres. Three-photon spectroscopy performed on a caesium-filled fibre detects Rydberg states up to a principal quantum number of n =40. Besides small energy-level shifts we observe narrow lines confirming the coherence of the Rydberg excitation. Using different Rydberg states and core diameters we study the influence of confinement within the fibre core after different exposure times. Understanding these effects is essential for the successful future development of novel applications based on integrated room temperature Rydberg systems. Hollow-core photonic crystal fibre (HC-PCF) has opened up new opportunities in the field of atomic spectroscopy, enabling both light and atoms to be confined in the same narrow channel over distances that exceed the Rayleigh length by many orders of magnitude [1] . Filled with alkali atoms, HC-PCF has been used to study low-lying excitations in ultracold alkali gases [2] as well as in thermal vapours [3] , [4] , [5] . Nonlinear optical experiments in particular benefit from the enhanced overlap between light and matter provided by HC-PCF, a recent example being the demonstration of all-optical switching by electromagnetically induced transparency using only a few hundred gating photons [2] , [3] , [4] . The use of kagome-style HC-PCF uniquely enables spectrally broadband transmission covering the wide range of optical wavelengths needed for Rydberg excitation schemes. The extreme polarizability of Rydberg states results in large mutual interactions that can provide even stronger optical nonlinearities [6] . This leads to strong dipole–dipole or van-der-Waals interactions [7] , which are effective over micron-scale distances even at room temperature [8] . One consequence of this is the Rydberg excitation blockade, which is the key element for controlled NOT gates [9] , [10] , single-photon sources [11] , [12] , antibunched [13] and attractive photons [14] , single-photon absorbers [15] and atom-light entanglement [16] . Every quantum optics experiment involving Rydberg states requires excellent control over the spatial arrangement of the atoms and the excitation light. Of particular interest is a configuration in which the blockade radius (typically a few microns) is larger than the width of the excitation volume, resulting in an effectively one-dimensional system. Such systems have recently been realized in free-space cold atom experiments, where the generation of anti-bunched [13] and attractive photons [14] has been successfully demonstrated. HC-PCF is a particularly suitable system [17] , especially for thermal atoms, as it provides optically accessible, easy-to-fill, micron-scale confinement volumes capable of withstanding corrosive alkali vapours. Additionally, the effective length of the one-dimensional system, which in free-space experiments is limited by diffraction, can be significantly increased. For successful integration of room temperature Rydberg systems into micron-scale devices, however, it is essential to understand how the Rydberg atoms are influenced by the nearby glass walls of the core [18] . While some effects, such as local fields created by adsorbed ions, mainly depend on the distance between the atom and the glass wall, other interactions are also affected by the thickness of the glass wall itself, for example, Casimir–Polder effects. These interactions are expected to be weaker in HC-PCF (compared to glass cells or capillaries) owing to the greatly reduced thickness of the glass walls surrounding the core (typically ~200 nm). Here we aim to demonstrate the feasibility of exciting Rydberg atoms inside a HC-PCF as well as reporting on the effects of confinement within the fibre core. As a result we have studied the influence of different core diameters and varying optical densities on a wide range of Rydberg states, so as to identify an optimal design for future integrated Rydberg systems based on HC-PCF. Experimental set-up In the experiments we used two different kagome-style HC-PCFs (kagome-PCFs), cleaved to lengths of ~13.5 cm and mounted in a UHV chamber, as shown in the experimental set-up in Fig. 1a . Scanning electron micrographs of the cross-sectional structure of both fibres are shown in Fig. 2 ; the core diameters are ~60 and ~19 μm. For the Rydberg spectroscopic measurements a coherent three-photon excitation scheme [19] involving lasers at 895, 1359 and 790 nm was chosen ( Fig. 1b ). The fibres were specifically selected to guide these wavelengths. All the beams were coupled into the fundamental mode of the fibre by focusing the light through UHV windows onto the fibre ends. 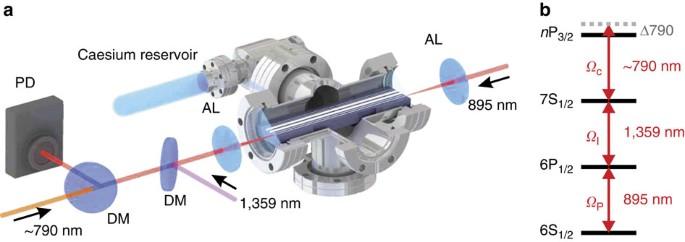Figure 1: Experimental set-up and excitation scheme. (a) A selection of kagome PCFs with different core diameters is mounted inside a vacuum chamber containing saturated caesium vapour. The three excitation beams are coupled into the fibre from both sides using achromatic lenses (AL). The beams are superimposed/separated using dichroic mirrors (DM), and the transmission of the counter-propagating 895 nm probe beam is measured at a photodiode (PD). (b) Three-photon excitation scheme up to a Rydberg level. The lasers driving the two lower transitions are locked on resonance while the Rydberg transition laser at 790 nm is scanned in frequency. Figure 1: Experimental set-up and excitation scheme. ( a ) A selection of kagome PCFs with different core diameters is mounted inside a vacuum chamber containing saturated caesium vapour. The three excitation beams are coupled into the fibre from both sides using achromatic lenses (AL). The beams are superimposed/separated using dichroic mirrors (DM), and the transmission of the counter-propagating 895 nm probe beam is measured at a photodiode (PD). ( b ) Three-photon excitation scheme up to a Rydberg level. The lasers driving the two lower transitions are locked on resonance while the Rydberg transition laser at 790 nm is scanned in frequency. 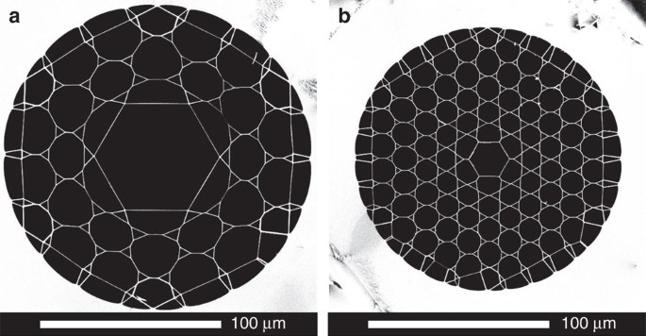Figure 2: Scanning electron micrographs of the two kagome PCFs studied. The special kagome-lattice cladding provides broadband transmission. The diameter of the hollow core region is ~60 μm for fibre (a) and ~19 μm for fibre (b). Full size image Figure 2: Scanning electron micrographs of the two kagome PCFs studied. The special kagome-lattice cladding provides broadband transmission. The diameter of the hollow core region is ~60 μm for fibre ( a ) and ~19 μm for fibre ( b ). Full size image The transmitted 895 nm signal served as a probe and its power was recorded by a photodiode. To compensate partly for the Doppler effect, the other two beams were launched into the fibre in the opposite direction. The polarization of all three beams was linear and parallel. The frequencies of the 895 and 1359, nm lasers were locked to sub-Doppler accuracy using a reference cell, while the laser driving the coupling transition at 790 nm was scanned in frequency. For comparison we always simultaneously recorded a reference spectrum in a conventional 5-mm-thick glass cell. The spectroscopy scheme was identical to that in the fibre. Three-photon Rydberg spectroscopy in a 60 μm core PCF As most of the properties of Rydberg atoms scale, in varying ways, with the principal quantum number n , we performed measurements at different values of n . A selection of the spectra obtained in the 60 μm core fibre is plotted in Fig. 3b,c along with the reference signal ( Fig. 3a ). The principal quantum number n of the excited Rydberg states (all of them of type n P 3/2 ) was varied between 26 and 40. To correct for the influence of the inner electrons, which are absent in a hydrogen atom, n is replaced by the effective principal quantum number n *= n − δ P , where δ P =3.558 is the quantum defect [20] . The origin of the frequency axis is determined by the reference signal position. To avoid any change in atomic density within one measurement series due to light-induced desorption [21] or heating of the fibre, the laser power was kept constant. As a consequence the observed coupling of the light fields to the Rydberg states decreased with increasing n *, resulting in a weaker signal. 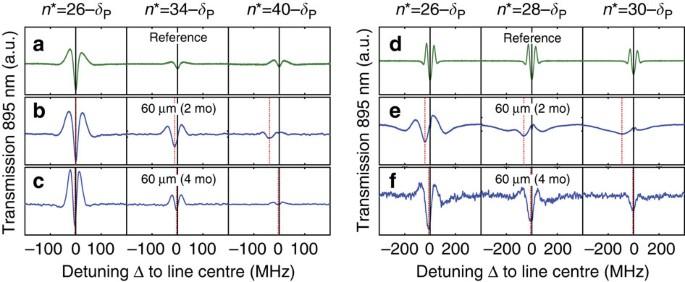Figure 3: Coherent three-photon spectroscopy for different Rydberg states. Transmission spectra of the probe light for the reference cell (aandd), defining the origin of the frequency axes (solid black line), and in fibre after a 2- (bande) and 4-month (candf) exposure to caesium, leading to different ODs. The signal is shown for three different principal quantum numbersn*=n−δPin a 60 μm core (bandc) and a 19 μm core (eandf) kagome PCF. The decreasing signal strength for higher values ofnoriginates from a decrease in the magnitude of the dipole matrix elements. The measured OD values are 0.4/2.9 for the 60 μm core fibre and 0.2/1.5 for the 19 μm core fibre after a 2-/4-month exposure. For the lower OD values and highern, a frequency shift in both fibres, and broadening of the signal in the 19 μm fibre relative to the reference cell signal are observed. We attribute these effects to background electric fields. The extracted signal positions are indicated by dotted red lines. For the higher OD values, after 4-month exposure, these effects are strongly reduced, resulting in a narrower line shape in case of the 19 μm core fibre and a vanishing of the redshift in both fibres. All measurement parameters are given in the Methods section. Figure 3: Coherent three-photon spectroscopy for different Rydberg states. Transmission spectra of the probe light for the reference cell ( a and d ), defining the origin of the frequency axes (solid black line), and in fibre after a 2- ( b and e ) and 4-month ( c and f ) exposure to caesium, leading to different ODs. The signal is shown for three different principal quantum numbers n* = n−δ P in a 60 μm core ( b and c ) and a 19 μm core ( e and f ) kagome PCF. The decreasing signal strength for higher values of n originates from a decrease in the magnitude of the dipole matrix elements. The measured OD values are 0.4/2.9 for the 60 μm core fibre and 0.2/1.5 for the 19 μm core fibre after a 2-/4-month exposure. For the lower OD values and higher n , a frequency shift in both fibres, and broadening of the signal in the 19 μm fibre relative to the reference cell signal are observed. We attribute these effects to background electric fields. The extracted signal positions are indicated by dotted red lines. For the higher OD values, after 4-month exposure, these effects are strongly reduced, resulting in a narrower line shape in case of the 19 μm core fibre and a vanishing of the redshift in both fibres. All measurement parameters are given in the Methods section. Full size image The measurements inside the fibre were carried out at different optical densities, in this case defined as OD=–ln( I out / I in ) at the D1 line ( F =3 to F ′=4) resonance. The optical density was calculated to be OD=0.4 for the measurement series in Fig. 3b and OD=2.9 for Fig. 3c , respectively (see Methods). Since both experiments were carried out at room temperature we mainly attribute this difference to the longer exposure time to the caesium vapour (4 months in Fig. 3c compared to 2 months in Fig. 3b ). However, between these two experiments the fibres were also subject to higher temperatures and strong light fields, which might also have influenced the atomic density in the core. The strongest deviation between the reference and the fibre signal is observed for high n* at the smaller OD ( Fig. 3b right-hand side), where the signal position is clearly shifted to lower frequencies, indicating that the Rydberg states are influenced by the confined environment. This frequency shift is, however, not present at higher optical density as shown in Fig. 3c for OD=2.9. This OD value is comparable to the one measured through the surrounding chamber (OD≈2.4). We therefore conclude that the system has reached equilibrium, that is, the fibre core is homogeneously filled. Nonetheless, it remains unclear what caused the line shifts in the first place and why they finally disappeared at higher OD values. To obtain a better understanding of possible influences on the Rydberg atoms we systematically measured this signal shift for a larger set of Rydberg states. In Fig. 4 the frequency shift between the signal inside the 60 μm fibre (blue squares) and the reference signal position is plotted versus the effective quantum number n * for optical densities 0.4 (filled blue squares) and 2.9 (open blue squares). For the lower OD value a clear shift is observable, increasing for higher n *. To identify the origin of this shift δ it is useful to compare its behaviour with well-known scaling laws for Rydberg atoms ( n *) m (ref. 22 ). Fitting the experimental data to a power law as shown in the log–log scaled inset in Fig. 4 results in m =6.7±0.7 (solid blue line). Since the polarizability α of Rydberg atoms scales with m =7, we are confident that the shift in the 60 μm is predominantly caused by static electric fields. By interpolating known values of polarizabilities for caesium P 3/2 Rydberg states [23] we estimate the field strength, using δ = αE 2 /2, to be ≈0.5 V cm −1 (Methods). 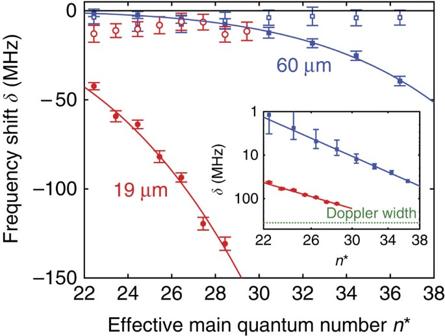Figure 4: Signal shift inside the fibre. The frequency shifts between the fibre and reference cell signal are shown as a function of the effective main quantum number for the 60 μm fibre (blue squares) and the 19 μm core fibre (red circles). The measurements were performed at exposure times of 2 months (filled) and ~4 months (open), resulting in ODs of 0.4/2.9 in the 60 μm fibre and 0.2/1.5 in the 19 μm fibre. Fitting the shift observable after 2 months of exposure time to the power lawδ~(n*)mleads tom=6.7±0.7 for the 60 μm core fibre andm=4.4±0.4 for the 19 μm core fibre plotted on a log–log scale in the inset where the Doppler line width is indicated by the horizontal dashed line for comparison. Figure 4: Signal shift inside the fibre. The frequency shifts between the fibre and reference cell signal are shown as a function of the effective main quantum number for the 60 μm fibre (blue squares) and the 19 μm core fibre (red circles). The measurements were performed at exposure times of 2 months (filled) and ~4 months (open), resulting in ODs of 0.4/2.9 in the 60 μm fibre and 0.2/1.5 in the 19 μm fibre. Fitting the shift observable after 2 months of exposure time to the power law δ ~( n *) m leads to m =6.7±0.7 for the 60 μm core fibre and m =4.4±0.4 for the 19 μm core fibre plotted on a log–log scale in the inset where the Doppler line width is indicated by the horizontal dashed line for comparison. Full size image In contrast, this shift was not observable at higher OD values, even for high values of n , which implies that static electric fields are no longer present in the inner core after 4 months. Three-photon Rydberg spectroscopy in a 19 μm core PCF Additionally we investigated the influence of a reduced mean distance between the Rydberg atoms and glass walls by measuring in a fibre with a reduced core diameter of 19 μm. The spectroscopy signals for three different principal quantum numbers n are shown in Fig. 3d–f . For the lower OD of 0.2, after a 2-month exposure to caesium a broadening of the line as well as a frequency redshift could be observed ( Fig. 3e ), both increasing with higher n . This redshift is up to ten times larger than the one measured in the 60 μm core fibre (filled-in red circles in Fig. 4 ). The fitted power law shown in the inset yields m =4.4±0.4 (solid red line). This shift does not match the scaling behaviour for a homogeneous electric field, indicating that inhomogeneous components or additional effects need to be considered. Inhomogeneous electric fields may also explain the broadening of the signal. It is important to point out that, in all measurements the frequency shift of the signal is smaller than the FWHM Doppler line width of ≈360 MHz represented by the horizontal dashed line in the inset in Fig. 4 . This indicates that all the measurements are dominated by coherent processes. After 4 months of exposure to caesium vapour, the OD in the 19 μm fibre core increased to 1.5 (compared to 2.4 in the surrounding chamber). A possible reason for this low value is that due to the smaller core size and therefore longer diffusion time, a full equilibrium had not yet been reached. Interestingly, the redshift that was observed after 2 months of exposure could no longer be observed after 4 months, even for high n * (open red circles in Fig. 4 ). Furthermore, the line width of the signal is reduced considerably ( Fig. 3f ), indicating that the influence of the confining core walls is smaller. This suggests that the dominant effect on the atoms, which we believe to be electric fields, was similar in both fibres. The disappearance of the frequency shifts after 4 months may perhaps be explained by a decrease in the nearby charge density or by the formation of a homogeneous layer of adsorbed caesium atoms on the core surface, which would shield the atoms from any electric fields. The fact that the frequency shifts could be significantly reduced by operating at higher values of OD is important for practical applications. The results demonstrate that the spectroscopy of Rydberg states inside HC-PCF is currently not fundamentally limited by interactions with the confining core walls. If the goal of a truly one-dimensional system is to be approached, however, even smaller core sizes are required, making it likely that line shifts (due to resonant or off-resonant coupling to the walls) will reappear, especially if higher-excited Rydberg states are to be explored. Therefore further systematic measurements, in combination with improved spectroscopic resolution, will be required to investigate these regimes and gain a more complete understanding of confined Rydberg atoms. Nevertheless, the results presented here are already highly promising, opening up various possibilities. For example, the selective excitation of higher-order modes [24] in fibre will allow atoms to be probed at different distances from the core walls. Higher-order modes, such as LG 10 , can also provide even tighter radial confinement of the light field, permitting the diameter of a blockaded system to be further reduced towards a genuinely one-dimensional system. In addition, Rydberg gases in the non-interacting regime could be used in many interesting applications. For example, fibre-based spectroscopy cells could be used as non-invasive microscopic microwave detectors [25] . Additional functionality could be achieved by incorporating gold nanowires [26] into the fibres, either to enable direct detection of the Rydberg population via a current [27] , or to frequency-modulate the probe light [28] at extremely low electric fields. Ultimately, splicing atom-filled HC-PCF to endlessly single-mode optical fibres may enable systems based on Rydberg atoms to be integrated into fibre-coupled devices operating at room temperature [29] . OD measurement The optical depth inside the fibre was calculated by an absorption measurement of the 895 nm light scanning the D1 line. To ensure that the spectroscopy signal was dominated by atoms inside the hollow core the absorption signal with 895 nm light coupled into the fundamental core mode was compared to the situation where the 895 nm light was coupled into the glass cladding. Since the ODs measured when light is coupled into the cladding are at least one order of magnitude smaller this assumption is valid. To extract the final in-core ODs the cladding values were subtracted from the core values. Laser and lock-in set-up The laser systems for 895 and 1.359 nm light were frequency locked to the 6S 1/2 →6P 1/2 transition (D1 line) by Doppler-free spectroscopy and to the 6P 1/2 →7S 1/2 transition by polarization spectroscopy. The three beams were superimposed using dichroic mirrors and launched into the kagome-PCF with achromatic lenses. The typical signal strength is of order 1% of the transmitted probe light without any amplification. To achieve a better signal-to-noise ratio a lock-in amplifier was used. To this end, in the first measurement series (2 months diffusion time) the 1,359 nm light was modulated at 1.1 kHz by a chopper wheel. To ensure that the OD of the system is not modulated in the same way by the 1,359 nm light, due to the effect of light-induced atomic desorption (LIAD), additional absorption measurements were performed. Because of its low intensity this beam did not show LIAD effects. In the second series of measurements (four months diffusion time) the 790 nm light was modulated instead. The intensity of this beam is much higher, but further absorption measurements showed that by modulating it much faster (50 kHz via an acousto-optic modulator) LIAD effects were greatly suppressed and could be neglected. Finally, identical spectroscopic measurements in the absence of any lock-in scheme showed that the results were not influenced by the measurement procedure. Coupling efficiencies and intensities The launch efficiency into the fibre was optimized both by imaging the mode profile at the end of the fibre and by maximizing the transmitted power. In this way we ensured that most of the light was coupled into the fundamental fibre mode for all beams. Experimental launch efficiencies of ~30% (1359, nm), ~40% (895 nm) and ~60% (790 nm) were achieved for the 60 μm core, and ~20% (1359, nm), ~30% (895 nm) and ~40% (790 nm) for the 19 μm core. These values include transmission losses in the fibre and the glass windows. The input powers in the first measurement series (after 2 months diffusion time) for the 60 μm (19 μm) fibre were P P =0.15 μW (0.3 μW) for the 895 nm probe beam, P I =7.0 μW (6.0 μW) for the 1359, nm intermediate beam and P C =70 mW (50 mW) for the 790 nm coupling beam. For the measurement series after 4 months diffusion the values were P P =0.5 μW (0.15 μW), P I =10.0 μW (10.0 μW) and P C =30 mW (20 mW) for the 60 μm (19 μm) fibre. For the measurements in the reference cell shown in Fig. 3 the adjusted powers were P P =2 μW, P I =200 μW and P C =20 mW, and the beam radii were w P =41.1±1.0 μm, w I =64.3±1.2 μm and w C =46.3±1.6 μm. The signals are averaged between 100 and 300 times. Transit time The 1/ e 2 beam radius w in the fibre core was calculated to be ~20 μm for the 60 μm core fibre and ~6 μm for the 19 μm core fibre. The transit-time broadening for the different systems can be calculated [30] by Γ tt =( v / w ) × (2 ln 2) −1/2 (where v is the atomic velocity) to be 2 π × 0.7 s −1 for the reference cell, 2 π × 1.5 s −1 for the 60 μm core fibre and 2 π × 4.9 s −1 for the 19 μm core fibre. Since the spectral width of the three-photon signal is between 15 and 50 MHz, depending on core diameter and quantum number, we were not limited by transit-time effects. This broadening mechanism will however become more important when the core size is further reduced. Data evaluation The raw data were evaluated as follows: The relative frequency change of the coupling laser ( x -axis in Fig. 3 ) was measured using a Fabry–Pérot interferometer. The detuning zero was extracted by fitting a quadratic function to the absorption dip at line centre in the reference signal. The central frequency of the fibre signal was located in the same manner. Since only the fibre signal was fed through a lock-in amplifier, it was necessary to consider the time delay in the electronics, which will translate into a constant offset frequency shift between the fibre and reference signal. This delay was measured to be ~8.0 ms for the first measurement series and ~400 μs for the second, depending on the different integration times. In future experiments both signals will be fed through a lock-in amplifier of the same type. Note that in Fig. 3e there are actually two signals overlapping. The small and narrow signal at the origin is due to atoms between the fibre ends and the windows. The overlapping of this signal with the reference position indicates that the offset calculations are in the correct range. The error bars on the frequency shift in Fig. 4 include the uncertainty in the lock-in amplifier delay, the uncertainty in scaling the frequency axis and uncertainties in fitting the line centres. How to cite this article: Epple, G. et al . Rydberg atoms in hollow-core photonic crystal fibres. Nat. Commun. 5:4132 doi: 10.1038/ncomms5132 (2014).